Rheb activation disrupts spine synapse formation through accumulation of syntenin in tuberous sclerosis complex Rheb is a small GTP-binding protein and its GTPase activity is activated by the complex of Tsc1 and Tsc2 whose mutations cause tuberous sclerosis complex (TSC). We previously reported that cultured TSC neurons showed impaired spine synapse morphogenesis in an mTORC1-independent manner. Here we show that the PDZ protein syntenin preferentially binds to the GDP-bound form of Rheb. The levels of syntenin are significantly higher in TSC neurons than in wild-type neurons because the Rheb-GDP-syntenin complex is prone to proteasomal degradation. Accumulated syntenin in TSC neurons disrupts spine synapse formation through inhibition of the association between syndecan-2 and calcium/calmodulin-dependent serine protein kinase. Instead, syntenin enhances excitatory shaft synapse formation on dendrites by interacting with ephrinB3. Downregulation of syntenin in TSC neurons restores both spine and shaft synapse densities. These findings suggest that Rheb-syntenin signalling may be a novel therapeutic target for abnormalities in spine and shaft synapses in TSC neurons. Dendritic spine formation and synaptogenesis are often preceded by a period in which numerous elongated filopodia extend from developing dendrites. The impairment in the conversion of filopodia to dendritic spines may lead to childhood cognitive disorders [1] . Synaptic abnormalities in neurodevelopmental disorders may be caused by mutations that affect synaptic proteins. For example, mutations in fmr1 , identified in fragile X syndrome, alter the properties of the FMRP protein, resulting in spine dysmorphogenesis [2] . The E3 ubiquitin ligase Ube3A, linked to Angelman syndrome, also controls spine formation [3] . Moreover, another autism-related protein neurobeachin regulates spine density and shaft synapse formation [4] . Thus, childhood mental disorders may be accompanied by morphological abnormalities of excitatory spine and/or shaft synapses. Tuberous sclerosis complex (TSC) is a systemic genetic disease that causes the growth of hamartomas in the brain and other organs [5] . The neuropsychiatric symptoms of TSC patients include intellectual disability, epilepsy and/or autism [5] . TSC results from inactivating mutations in either Tsc1 (ref. 6 ) or Tsc2 (ref. 7 ), which encode hamartin and tuberin, respectively. Hamartin and tuberin form a complex that exhibits guanosine triphosphatase (GTPase)-activating protein activity towards the small GTP-binding protein Rheb [8] , [9] , [10] . Inactivating mutations in Tsc1 or Tsc2 result in the accumulation of the GTP-bound form of Rheb, which activates mammalian target of rapamycin complex 1 (mTORC1; ref. 11 ). A Golgi study of surgical specimens from a TSC patient reported that cortical neurons showed aberrant spine development [12] . Several lines of evidence also suggest that Tsc1 +/− or Tsc2 +/− rodents show impairments in dendritic spine formation [13] , [14] and cognitive behaviours [15] , suggesting that the activation of mTORC1 in TSC neurons may cause memory disturbances, likely through dendritic spine abnormalities. However, the mTORC1 signalling pathway has been shown to be activated during learning and is required for spatial memory formation [16] . This discrepancy may indicate that an mTORC1-independent mechanism may be involved in memory impairments in TSC. Syndecan-2 is a transmembrane heparan sulphate proteoglycan that promotes spine formation [16] , [17] , [18] . The C-terminal EFYA motif of syndecan-2 is necessary for dendritic spinogenesis, and this motif binds to the PSD-95, Dlg and ZO1 (PDZ) domains of calcium/calmodulin-dependent serine protein kinase (CASK). CASK is known to associate with F-actin via its binding to protein 4.1 (ref. 18 ), and it may mediate spine morphogenesis through syndecan-2. However, the C terminus of syndecan-2 also binds to syntenin, a scaffold protein with two PDZ domains [19] . In contrast to CASK, overexpression of syntenin in hippocampal neurons increases filopodia-like dendritic protrusions [20] , suggesting that syntenin competes with CASK for syndecan-2. In the present study, we propose a novel mechanism for dendritic spine morphogenesis. We previously showed that activation of Rheb, but not mTORC1, impaired spine synapse formation in TSC neurons [14] . To further elucidate this mechanism, we sought to detect a new Rheb-mediated signalling pathway in the brain and to identify syntenin as a novel Rheb-binding protein. Syntenin preferentially binds to the GDP form of Rheb, and this complex is prone to proteasomal degradation in wild-type (WT) neurons. The consequent reduction in syntenin levels allows CASK to associate with syndecan-2, leading to stabilization of spine structure. In Tsc2 +/− neurons, the syntenin released from Rheb-GTP associates with syndecan-2, resulting in decreased spine synapse density. Syntenin also interacts with ephrinB3 and increases the density of excitatory shaft synapses. In fact, downregulation of syntenin restores spine and shaft synapse densities in Tsc2 +/− neurons. These results suggest that syntenin is a regulator of spine and shaft synapse density, and link syntenin to a novel pathophysiological mechanism implicated in neurodevelopmental disorders. Rheb associates with syntenin We previously reported that dendritic spine synapse density was decreased in TSC neurons through an mTOR-independent mechanism [14] . We found that activation of Rheb, but not mTORC1, reduced spine synapse density, and the expression of a dominant-negative form of Rheb or treatment with farnesyl transferase inhibitors largely restored spine synapse density in Tsc2 +/− neurons. These results suggest that the mTOR-independent mechanism controlling spine synapse density involves Rheb, and that this mechanism may be dysregulated in TSC neurons. To elucidate this mechanism, in this study, we searched for a Rheb-associating protein using the yeast two-hybrid system. We identified a PDZ domain-containing scaffold protein, syntenin [19] , as a novel Rheb-binding partner. The potential interaction between Rheb and syntenin was confirmed by co-immunoprecipitation of Rheb with syntenin from rat brain lysates ( Fig. 1a ). Furthermore, Rheb D60I protein was pulled down with glutathione S-transferase (GST)-fused syntenin ( Fig. 1b ). The association of syntenin with Rheb appeared to depend on the nucleotide-binding state of Rheb, as the GDP-bound form (Rheb D60I ) exhibited a significantly stronger binding to syntenin than did the GTP-bound form (Rheb Q64V ; Fig. 1c,d ). 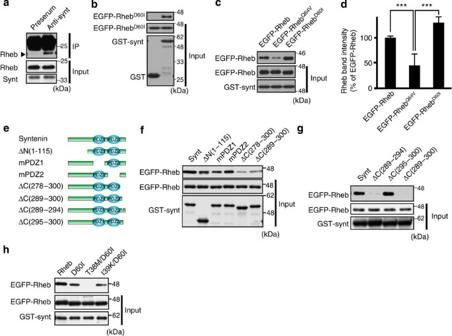Figure 1: Rheb associates with syntenin. (a) Rat brain lysates were immunoprecipitated (IP) with preimmune serum (preserum, lane 1) or anti-syntenin (synt) antibody (lane 2). Rheb in the precipitates was detected using immunoblotting. (b) Pull-down of RhebD60Iwith GST-syntenin, not with GST alone, from EGFP-RhebD60I-expressing HEK293T cells. (c) GDP-dependent binding of Rheb to syntenin. EGFP-Rheb-, RhebD60I- or RhebQ64V-expressing cell lysates were precipitated with GST-syntenin. The precipitates were immunoblotted with anti-GFP antibody. (d) Quantification of EGFP-Rheb pulled down with GST-syntenin as shown inc(n=8 independent experiments, ***P<0.001, unpaired, two-tailedt-test). (e) Schematic diagram of WT syntenin and varioussynteninmutants: N-terminal domain-deleted (ΔN(1–115)), PDZ1 domain-mutated (mPDZ1), PDZ2 domain-mutated (mPDZ2) and C-terminal domain-deleted (ΔC(278–300),ΔC(289–300),ΔC(289–294)andΔC(295–300)). (f,g) Identification of the Rheb-binding domain of syntenin. Each syntenin mutant fused to GST was examined for binding to RhebD60Iin HEK293T cells using pull-down assays. (h) RhebD60I, RhebT38M/D60Ior RhebI39K/D60Imutants expressed in HEK293T cells were examined for binding to GST-syntenin using pull-down assays. Blots ina–c,f–h) are cropped and full-length blots are presented inSupplementary Fig. 6a–f. All data are presented as mean±s.e.m. Figure 1: Rheb associates with syntenin. ( a ) Rat brain lysates were immunoprecipitated (IP) with preimmune serum (preserum, lane 1) or anti-syntenin (synt) antibody (lane 2). Rheb in the precipitates was detected using immunoblotting. ( b ) Pull-down of Rheb D60I with GST-syntenin, not with GST alone, from EGFP-Rheb D60I -expressing HEK293T cells. ( c ) GDP-dependent binding of Rheb to syntenin. EGFP-Rheb-, Rheb D60I - or Rheb Q64V -expressing cell lysates were precipitated with GST-syntenin. The precipitates were immunoblotted with anti-GFP antibody. ( d ) Quantification of EGFP-Rheb pulled down with GST-syntenin as shown in c ( n =8 independent experiments, *** P <0.001, unpaired, two-tailed t -test). ( e ) Schematic diagram of WT syntenin and various syntenin mutants: N-terminal domain-deleted ( ΔN(1–115) ), PDZ1 domain-mutated ( mPDZ1 ), PDZ2 domain-mutated ( mPDZ2 ) and C-terminal domain-deleted ( ΔC(278–300) , ΔC(289–300) , ΔC(289–294) and ΔC(295–300) ). ( f , g ) Identification of the Rheb-binding domain of syntenin. Each syntenin mutant fused to GST was examined for binding to Rheb D60I in HEK293T cells using pull-down assays. ( h ) Rheb D60I , Rheb T38M/D60I or Rheb I39K/D60I mutants expressed in HEK293T cells were examined for binding to GST-syntenin using pull-down assays. Blots in a – c , f – h ) are cropped and full-length blots are presented in Supplementary Fig. 6a–f . All data are presented as mean±s.e.m. Full size image We localized the Rheb-binding region of syntenin to its C-terminal segment but not to either PDZ domain because the affinity of Rheb to syntenin was significantly reduced by the C-terminal deletions (Δ278–300 and Δ289–300) but not by the mPDZ1 or mPDZ2 (ref. 19 ; Fig. 1e,f ). Furthermore, syntenin ΔC(289–294) showed no interaction with Rheb ( Fig. 1g ), indicating that the Rheb-binding region of syntenin is localized between residues 289 and 294. Conversely, syntenin interacted with the switch I region (also called the effector region) of Rheb in pull-down experiments. Specifically, a T38M, but not I39K, mutation in Rheb D60I reduced the binding to syntenin ( Fig. 1h ), suggesting that residues exposed only in Rheb-GDP form may mediate the binding of the two proteins [21] . Syntenin regulates dendritic spine synapse density To elucidate the role of the Rheb-syntenin interaction in spine synapse morphogenesis, we first compared syntenin levels in WT and TSC neurons. We used spontaneous Tsc2 -mutated rats (Eker) as a model of TSC [22] . We cultured hippocampal neurons of WT and heterozygous Eker ( Tsc2 +/– ) rat embryos, fixed the cultures at 21 days in vitro (DIV) and immunostained the neurons with anti-syntenin antibody. As shown in Fig. 2a,b , syntenin levels were significantly higher in Tsc2 +/− neurons than in WT neurons. This result was consistent with an increase in syntenin levels in Tsc2 +/− brains compared with those in WT brains ( Fig. 2c,d ), suggesting that the Tsc2 mutation may affect neuronal syntenin levels, possibly via Rheb. 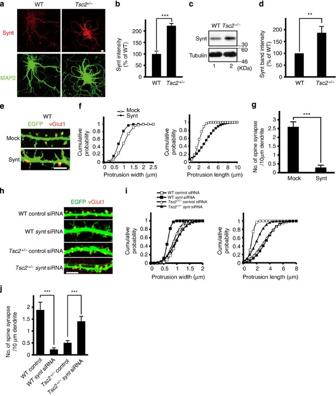Figure 2: Syntenin negatively regulates spine synapse formation. (a) Immunostaining of WT (left) andTsc2+/−(right) neurons using anti-syntenin (anti-synt; top) and MAP2 (bottom) antibodies. Scale bar, 10 μm. (b) Quantification of the syntenin immunoreactivity as shown ina, normalized to that of MAP2 (n=5/3 (WT), 6/3 (Tsc2+/−) (DIV 16) neurons/experiments; ***P<0.001, unpaired, two-tailedt-test). (c) Levels of syntenin and tubulin in WT (lane 1) andTsc2+/−rat brains (lane 2). These blots are cropped and full-length blots are presented inSupplementary Fig. 6g. (d) Quantification of syntenin levels inTsc2+/−rat brains normalized to WT levels (n=8 independent experiments, **P<0.01, unpaired, two-tailedt-test). (e) Dendrites of EGFP- and mock- (upper) or ECFP-syntenin (synt)-expressing (lower) WT neurons at DIV 21. The neurons were immunolabelled with anti-vGlut1. Scale bar, 10 μm. (f) Cumulative probability distributions of the protrusion width and length as shown ine. The syntenin-expressing neurons demonstrate narrower (D=0.3596,P<0.001) and longer (D=0.3623,P<0.001) dendritic protrusions than mock transfectants (Kolmogorov–Smirnov test). (g) Quantification of vGlut1-positive spine synapse density in the neurons transfected as ine. In total, 496/5/3 (mock) and 568/6/3 (syntenin) protrusions/neurons/experiments, respectively, were analysed (***P<0.001, two-tailedt-test). (h) Dendrites of WT andTsc2+/−neurons transfected withsynteninsiRNA or scrambled siRNA. Scale bar, 10 μm. (i) Cumulative probability plots of the protrusion width and length as shown inh.SynteninsiRNA-expressingTsc2+/−neurons show wider (D=0.1253,P<0.001) and shorter (D=0.3474,P<0.001) dendritic protrusions than scrambled siRNA (Kolmogorov–Smirnov test). (j) Quantitative analysis of the spine synapse densities as shown inh(n=500/5/3 (WT,synteninsiRNA), 500/5/3 (WT, scrambled siRNA), 1,034/10/5 (Tsc2+/−,synteninsiRNA) and 1,146/10/5 (Tsc2+/−, scrambled siRNA) protrusions/neurons/experiments, ***P<0.001, two-way analysis of variance, (ANOVA)post hocTukey test). All data are presented as mean±s.e.m. Figure 2: Syntenin negatively regulates spine synapse formation. ( a ) Immunostaining of WT (left) and Tsc2 +/− (right) neurons using anti-syntenin (anti-synt; top) and MAP2 (bottom) antibodies. Scale bar, 10 μm. ( b ) Quantification of the syntenin immunoreactivity as shown in a , normalized to that of MAP2 ( n =5/3 (WT), 6/3 ( Tsc2 +/− ) (DIV 16) neurons/experiments; *** P <0.001, unpaired, two-tailed t -test). ( c ) Levels of syntenin and tubulin in WT (lane 1) and Tsc2 +/− rat brains (lane 2). These blots are cropped and full-length blots are presented in Supplementary Fig. 6g . ( d ) Quantification of syntenin levels in Tsc2 +/− rat brains normalized to WT levels ( n =8 independent experiments, ** P <0.01, unpaired, two-tailed t -test). ( e ) Dendrites of EGFP- and mock- (upper) or ECFP-syntenin (synt)-expressing (lower) WT neurons at DIV 21. The neurons were immunolabelled with anti-vGlut1. Scale bar, 10 μm. ( f ) Cumulative probability distributions of the protrusion width and length as shown in e . The syntenin-expressing neurons demonstrate narrower ( D =0.3596, P <0.001) and longer ( D =0.3623, P <0.001) dendritic protrusions than mock transfectants (Kolmogorov–Smirnov test). ( g ) Quantification of vGlut1-positive spine synapse density in the neurons transfected as in e . In total, 496/5/3 (mock) and 568/6/3 (syntenin) protrusions/neurons/experiments, respectively, were analysed (*** P <0.001, two-tailed t -test). ( h ) Dendrites of WT and Tsc2 +/− neurons transfected with syntenin siRNA or scrambled siRNA. Scale bar, 10 μm. ( i ) Cumulative probability plots of the protrusion width and length as shown in h . Syntenin siRNA-expressing Tsc2 +/− neurons show wider ( D =0.1253, P <0.001) and shorter ( D =0.3474, P <0.001) dendritic protrusions than scrambled siRNA (Kolmogorov–Smirnov test). ( j ) Quantitative analysis of the spine synapse densities as shown in h ( n =500/5/3 (WT, syntenin siRNA), 500/5/3 (WT, scrambled siRNA), 1,034/10/5 ( Tsc2 +/− , syntenin siRNA) and 1,146/10/5 ( Tsc2 +/− , scrambled siRNA) protrusions/neurons/experiments, *** P <0.001, two-way analysis of variance, (ANOVA) post hoc Tukey test). All data are presented as mean±s.e.m. Full size image To test whether the nucleotide-binding state of Rheb regulates syntenin levels, we overexpressed the GTP-bound form of Rheb (Rheb Q64V ) in cultured hippocampal neurons [14] . The expression of active Rheb significantly increased both the somatic and dendritic levels of syntenin in hippocampal neurons compared with adjacent untransfected neurons ( Supplementary Fig. 1a,b ). By contrast, the expression of Rheb D60I decreased syntenin levels in cultured neurons ( Supplementary Fig. 1c,d ). These results suggest that the nucleotide-binding state of Rheb controls the syntenin levels in hippocampal neurons. To confirm the effects of neuronal syntenin levels on spine and synapse formation, we overexpressed or knocked down syntenin in primary cultures of hippocampal neurons. Overexpression of syntenin in WT neurons decreased and increased dendritic protrusion width and length, respectively ( Fig. 2e,f ). Furthermore, syntenin expression drastically reduced spine synapse density ( Fig. 2e,g ), as observed previously in Rheb Q64V -expressing WT neurons or Tsc2 +/− neurons [14] . We then knocked down the endogenous syntenin levels in Tsc2 +/− neurons, whose syntenin levels were higher than those in WT neurons. Syntenin short interfering RNA (siRNA) reduced the expression of exogenous syntenin by 92.4% in HEK293T cells ( Supplementary Fig. 1e ). The transfection of syntenin siRNA into Tsc2 +/− neurons reduced the endogenous syntenin levels ( Supplementary Fig. 1f ) and induced wider and shorter dendritic protrusions ( Fig. 2h,i ). Syntenin knockdown also drastically enhanced spine synapse density in Tsc2 +/− neurons ( Fig. 2j ). Accordingly, a reduction in syntenin levels may restore spine synapse density in Tsc2 +/− neurons. By contrast, unexpectedly, knockdown of syntenin in WT neurons also disrupted spine synapse morphogenesis ( Fig. 2h,j ) and produced narrower and longer filopodia-like protrusions ( Fig. 2i ). Thus, both increasing and decreasing syntenin levels can affect spine synapse formation, suggesting that neuronal syntenin levels must be maintained within a narrow range for normal spine development. The Rheb-syntenin complex is degraded by proteasomes What mechanism underlies the increase in syntenin levels in TSC neurons? One possibility is the upregulation of syntenin production, and another is the inhibition of syntenin degradation. The former is unlikely because the mTORC1 inhibitor rapamycin failed to reduce syntenin levels in Tsc2 +/− neurons (unpublished observations). Recent work has demonstrated that the proteasome system regulates activity-dependent spine outgrowth [23] . Therefore, we assumed that syntenin levels may be regulated by the ubiquitin–proteasome system and that normal steady-state levels of syntenin degradation are required for spine synapse development. We treated Rheb D60I -expressing Tsc2 +/− neurons with the proteasomal inhibitors lactacystin (0.5 μM) or MG132 (0.1 μM) for 2 days, and observed that the Rheb D60I -induced decreases and increases in syntenin levels and spine synapse density, respectively, were prevented by either inhibitor ( Fig. 3a–d ; unpublished data). Proteasomal inhibitor alone did not change spine synapse density in WT neurons ( Fig. 3d ), consistent with a previous study [23] . Furthermore, knockdown of syntenin rescued spine synapse density in lactacystin-treated neurons ( Fig. 3c,d ). Thus, Rheb D60I -induced spine synapse morphogenesis in Tsc2 +/− neurons may be closely related to the reduction in syntenin levels by proteasomal degradation. 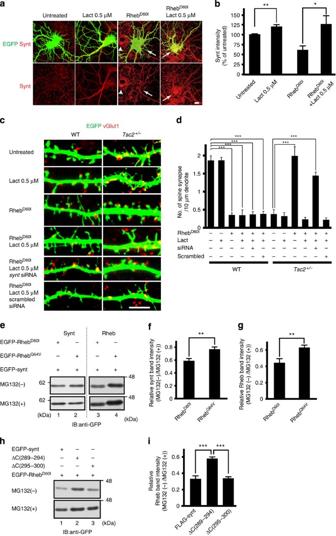Figure 3: Proteasomal degradation of the Rheb-syntenin complex is required for spine formation. (a) Treatment with lactacystin (Lact; 0.5 μM) for 2 days increased syntenin (synt) levels in WT and RhebD60I-expressedTsc2+/−neurons. Arrows and arrowheads indicate transfected and untransfected neurons, respectively. Scale bar, 10 μm. (b) Quantification of the syntenin levels as shown ina(n=10/3 neurons/experiments per condition, *P<0.05, **P<0.01, unpaired, two-tailedt-test). (c) Dendrites of untransfected,RhebD60I-transfected orRhebD60Iplus scrambled orsynteninsiRNA-transfected WT andTsc2+/−neurons treated or untreated with lactacystin. Scale bar, 10 μm. (d) Quantification of the spine synapse density as shown inc(n=500/5/3 (WT, untreated), 500/5/3 (WT, treated with 0.5 μM lactacystin), 500/5/3 (WT, RhebD60I), 500/5/3 (WT, RhebD60Itreated with 0.5 μM lactacystin), 500/5/3 (WT, RhebD60Itreated with 0.5 μM lactacystin+syntenin siRNA), 500/5/3 (WT, RhebD60Itreated with 0.5 μM lactacystin+scrambled siRNA), 500/5/3 (Tsc2+/−, untreated), 500/5/3 (Tsc2+/−, treated with 0.5 μM lactacystin), 1,029/10/5 (Tsc2+/−, RhebD60I), 1,017/10/5 (Tsc2+/−, RhebD60Itreated with 0.5 μM lactacystin), 500/5/3 (Tsc2+/−, RhebD60Itreated with 0.5 μM lactacystin+syntenin siRNA), 500/5/3 (Tsc2+/−, RhebD60Itreated with 0.5 μM lactacystin+scrambled siRNA) and protrusions/neurons/experiments, ***P<0.001, three-way ANOVA,post hocTukey test). (e) Left, western blots of syntenin (lanes 1 and 2) and Rheb (lanes 3 and 4) from untreated (top) and MG132-treated (bottom) COS-7 cells coexpressing EGFP-syntenin and EGFP-RhebD60Ior RhebQ64V. (f,g) Quantification of the relative syntenin (f) and Rheb (g) levels in the absence of MG132 compared with those in the presence of MG132 shown ine(n=8 independent experiments, **P<0.01, unpaired, two-tailedt-test). (h) Immunoblots (IB) of EGFP-Rheb from untreated (top) and MG132-treated (bottom) COS-7 cells expressing EGFP-RhebD60Iplus EGFP-syntenin (lane 1), synteninΔC(289–294)(lane 2) or synteninΔC(295–300)(lane 3). (i) Quantification of the relative Rheb levels with each syntenin mutant in the absence of MG132 compared with those in the presence of MG132 as shown inh(n=8 independent experiments, ***P<0.001, two-tailedt-test). Blots ine,hare cropped, and full-length blots are presented inSupplementary Fig. 6h,i. All data are presented as mean±s.e.m. Figure 3: Proteasomal degradation of the Rheb-syntenin complex is required for spine formation. ( a ) Treatment with lactacystin (Lact; 0.5 μM) for 2 days increased syntenin (synt) levels in WT and Rheb D60I -expressed Tsc2 +/− neurons. Arrows and arrowheads indicate transfected and untransfected neurons, respectively. Scale bar, 10 μm. ( b ) Quantification of the syntenin levels as shown in a ( n =10/3 neurons/experiments per condition, * P <0.05, ** P <0.01, unpaired, two-tailed t -test). ( c ) Dendrites of untransfected, Rheb D60I -transfected or Rheb D60I plus scrambled or syntenin siRNA-transfected WT and Tsc2 +/− neurons treated or untreated with lactacystin. Scale bar, 10 μm. ( d ) Quantification of the spine synapse density as shown in c ( n =500/5/3 (WT, untreated), 500/5/3 (WT, treated with 0.5 μM lactacystin), 500/5/3 (WT, Rheb D60I ), 500/5/3 (WT, Rheb D60I treated with 0.5 μM lactacystin), 500/5/3 (WT, Rheb D60I treated with 0.5 μM lactacystin+syntenin siRNA), 500/5/3 (WT, Rheb D60I treated with 0.5 μM lactacystin+scrambled siRNA), 500/5/3 ( Tsc2 +/− , untreated), 500/5/3 ( Tsc2 +/− , treated with 0.5 μM lactacystin), 1,029/10/5 ( Tsc2 +/− , Rheb D60I ), 1,017/10/5 ( Tsc2 +/− , Rheb D60I treated with 0.5 μM lactacystin), 500/5/3 ( Tsc2 +/− , Rheb D60I treated with 0.5 μM lactacystin+syntenin siRNA), 500/5/3 ( Tsc2 +/− , Rheb D60I treated with 0.5 μM lactacystin+scrambled siRNA) and protrusions/neurons/experiments, *** P <0.001, three-way ANOVA, post hoc Tukey test). ( e ) Left, western blots of syntenin (lanes 1 and 2) and Rheb (lanes 3 and 4) from untreated (top) and MG132-treated (bottom) COS-7 cells coexpressing EGFP-syntenin and EGFP-Rheb D60I or Rheb Q64V . ( f , g ) Quantification of the relative syntenin ( f ) and Rheb ( g ) levels in the absence of MG132 compared with those in the presence of MG132 shown in e ( n =8 independent experiments, ** P <0.01, unpaired, two-tailed t -test). ( h ) Immunoblots (IB) of EGFP-Rheb from untreated (top) and MG132-treated (bottom) COS-7 cells expressing EGFP-Rheb D60I plus EGFP-syntenin (lane 1), syntenin ΔC(289–294) (lane 2) or syntenin ΔC(295–300) (lane 3). ( i ) Quantification of the relative Rheb levels with each syntenin mutant in the absence of MG132 compared with those in the presence of MG132 as shown in h ( n =8 independent experiments, *** P <0.001, two-tailed t -test). Blots in e , h are cropped, and full-length blots are presented in Supplementary Fig. 6h,i . All data are presented as mean±s.e.m. Full size image To further elucidate the mechanism of syntenin downregulation, we investigated whether proteasomal degradation of syntenin depends on the nucleotide-binding state of Rheb. Syntenin was co-expressed with Rheb D60I or Rheb Q64V in COS-7 cells, which were treated with MG132 (ref. 24 ) or untreated. We compared the syntenin levels between MG132-treated and -untreated cells, and observed that the proteasomal degradation of syntenin was enhanced in the Rheb-GDP state compared with that in the Rheb-GTP state ( Fig. 3e,f ). Moreover, the GDP-bound form of Rheb was more sensitive to proteasomal degradation than Rheb-GTP ( Fig. 3e,g ). Next, we tested whether the association between syntenin and Rheb is required for the proteasomal degradation of both proteins. We co-expressed Rheb D60I with either intact syntenin or syntenin ΔC(289–294) , a mutant with a deletion of the Rheb-binding site, in COS-7 cells. Syntenin ΔC(289–294) drastically reduced the degradation of Rheb D60I ( Fig. 3h,i ), indicating that the proteasomal degradation of Rheb is enhanced by its interaction with syntenin. Syntenin competes with CASK for association with syndecan-2 To investigate the mechanism underlying the syntenin-induced decrease in spine synapse density, we identified the domain of syntenin that participates in this process. We created siRNA-resistant forms of N-terminal-deleted ( syntenin* ΔN(1–115) ), PDZ1-mutated ( syntenin* mPDZ1 ), PDZ2-mutated ( syntenin* mPDZ2 ) and C-terminal-deleted ( syntenin* ΔC(289–300) ) syntenin expression constructs. We co-transfected each syntenin mutant with syntenin siRNA to downregulate endogenous syntenin in primary neurons. Among the various syntenin mutants, only syntenin* mPDZ2 reversed the spine synapse density ( Supplementary Fig. 2a–c ), suggesting that the PDZ2 domain of syntenin mediates spine synapse dysmorphogenesis. The PDZ2 domain of syntenin has been associated with various proteins [25] . Of the more than 20 syntenin-binding proteins, only syndecan-2 has been demonstrated to regulate dendritic spine formation [17] , [18] , [26] . To clarify whether syndecan-2 is involved in aberrant spinogenesis in TSC neurons, we downregulated both syntenin and syndecan-2 in Tsc2 +/− neurons. Syndecan-2 siRNA reduced endogenous and exogenous syndecan-2 levels in cultured neurons and HEK293T cells, respectively ( Supplementary Fig. 2d,e ). Knockdown of syndecan-2 alone abolished normal spine synapse formation in WT neurons, confirming that syndecan-2 plays a crucial role in normal spine development. Similarly, syndecan-2 knockdown in Tsc2 +/− neurons did not restore spine formation, but concomitant reduction in syndecan-2 abolished the recovery of spine synapse density produced by syntenin siRNA ( Fig. 4a,b ). These results suggest that increased syntenin may disrupt spine synapse formation through association with syndecan-2. 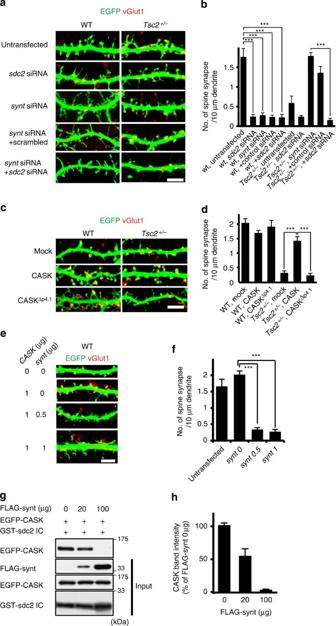Figure 4: Syntenin prevents spine formation by competing with CASK for binding to syndecan-2. (a) Dendrites of WT andTsc2+/−neurons either untransfected or transfected withsyndecan-2(sdc2) siRNA,syntenin(synt) siRNA,synteninsiRNA plus scrambled siRNA orsynteninsiRNA plussyndecan-2. Scale bar, 10 μm. (b) Quantification of spine synapse density as shown ina(n=500/5/3 (WT, untransfected), 500/5/3 (WT,syndecan-2siRNA), 500/5/3 (WT,synteninsiRNA), 500/5/3 (WT,synteninsiRNA+scrambled siRNA) and 500/5/3 (WT,synteninsiRNA+syndecan-2siRNA) protrusions/neurons/experiments, 500/5/3 (Tsc2+/−, untransfected), 500/5/3 (Tsc2+/−,syndecan-2siRNA), 500/5/3 (Tsc2+/−,synteninsiRNA), 893/10/5 (Tsc2+/−,synteninsiRNA+scrambled siRNA) and 1,196/10/5 (Tsc2+/−, synteninsiRNA+syndecan-2siRNA) protrusions/neurons/experiments, ***P<0.001, two-way ANOVA,post hocTukey test). (c) Dendrites of mock-, CASK- or CASKΔp4.1-transfected WT andTsc2+/−neurons. Scale bar, 10 μm. (d) Quantification of spine synapse density shown inc(n=500/5/3 (WT, mock), 500/5/3 (WT, CASK), 500/5/3 (WT, CASKΔp4.1), 1,023/10/5 (Tsc2+/−, mock), 1,070/10/5 (Tsc2+/−, CASK) 1,040/10/5 (Tsc2+/−, CASKΔp4.1) protrusions/neurons/experiments, ***P<0.001, unpaired, two-way ANOVA,post hocTukey test). (e) Dendrites of WT hippocampal neurons transfected withEGFPorEGFP-CASKplus 0, 0.5 or 1 μg ofECFP-synteninwere immunolabelled with anti-GFP and anti-vGlut1 antibodies. Scale bar, 10 μm. (f) Quantification of spine synapse densities as shown ine(n=500/5/3 (CASK 0, synt 0), 1,014/10/5 (CASK 1, synt 0), 953/10/5 (CASK 1, synt 0.5) and 1,152/10/5 (CASK 1, synt 1) protrusions/neurons/experiments, ***P<0.001, two-tailedt-test). (g) Pull-down assays showing that FLAG-syntenin inhibits the binding of EGFP-CASK to the IC of syndecan-2 (GST-sdc2 IC) in a dose-dependent manner. These blots are cropped and full-length blots are presented inSupplementary Fig. 6j. (h) Quantification of EGFP-CASK pulled down with GST-sdc2 IC in the presence of increasing amount of FLAG-syntenin (n=7 independent experiments). All data are presented as mean±s.e.m. Figure 4: Syntenin prevents spine formation by competing with CASK for binding to syndecan-2. ( a ) Dendrites of WT and Tsc2 +/− neurons either untransfected or transfected with syndecan-2 (sdc2) siRNA, syntenin (synt) siRNA, syntenin siRNA plus scrambled siRNA or syntenin siRNA plus syndecan-2 . Scale bar, 10 μm. ( b ) Quantification of spine synapse density as shown in a ( n =500/5/3 (WT, untransfected), 500/5/3 (WT, syndecan-2 siRNA), 500/5/3 (WT, syntenin siRNA), 500/5/3 (WT, syntenin siRNA+scrambled siRNA) and 500/5/3 (WT, syntenin siRNA+ syndecan-2 siRNA) protrusions/neurons/experiments, 500/5/3 ( Tsc2 +/− , untransfected), 500/5/3 ( Tsc2 +/− , syndecan-2 siRNA), 500/5/3 ( Tsc2 +/− , syntenin siRNA), 893/10/5 ( Tsc2 +/− , syntenin siRNA+scrambled siRNA) and 1,196/10/5 ( Tsc2 +/− , syntenin siRNA+ syndecan-2 siRNA) protrusions/neurons/experiments, *** P <0.001, two-way ANOVA, post hoc Tukey test). ( c ) Dendrites of mock-, CASK- or CASK Δp4.1 -transfected WT and Tsc2 +/− neurons. Scale bar, 10 μm. ( d ) Quantification of spine synapse density shown in c ( n =500/5/3 (WT, mock), 500/5/3 (WT, CASK), 500/5/3 (WT, CASK Δp4.1 ), 1,023/10/5 ( Tsc2 +/− , mock), 1,070/10/5 ( Tsc2 +/− , CASK) 1,040/10/5 ( Tsc2 +/− , CASK Δp4.1 ) protrusions/neurons/experiments, *** P <0.001, unpaired, two-way ANOVA, post hoc Tukey test). ( e ) Dendrites of WT hippocampal neurons transfected with EGFP or EGFP-CASK plus 0, 0.5 or 1 μg of ECFP-syntenin were immunolabelled with anti-GFP and anti-vGlut1 antibodies. Scale bar, 10 μm. ( f ) Quantification of spine synapse densities as shown in e ( n =500/5/3 (CASK 0, synt 0), 1,014/10/5 (CASK 1, synt 0), 953/10/5 (CASK 1, synt 0.5) and 1,152/10/5 (CASK 1, synt 1) protrusions/neurons/experiments, *** P <0.001, two-tailed t -test). ( g ) Pull-down assays showing that FLAG-syntenin inhibits the binding of EGFP-CASK to the IC of syndecan-2 (GST-sdc2 IC) in a dose-dependent manner. These blots are cropped and full-length blots are presented in Supplementary Fig. 6j . ( h ) Quantification of EGFP-CASK pulled down with GST-sdc2 IC in the presence of increasing amount of FLAG-syntenin ( n =7 independent experiments). All data are presented as mean±s.e.m. Full size image Similar to syntenin, CASK interacts with the C-terminal EFYA motif of syndecan-2 and promotes dendritic spine maturation [16] , [27] . We examined whether the binding of syndecan-2 to CASK and syntenin is mutually exclusive. We first tested the ability of CASK to induce spine synapse formation. The overexpression of CASK in Tsc2 +/− neurons also increased spine synapse density as well as syntenin knockdown ( Fig. 4c,d ); however, syntenin levels were not changed by CASK expression ( Supplementary Fig. 2f,g ), suggesting that an increase in CASK relative to syntenin restores spine synapse formation in Tsc2 +/− neurons. Further increases in syntenin impaired the ability of CASK to enhance spine synapse formation ( Fig. 4e,f ). We then examined whether the inhibitory effects of syntenin reflect competition between CASK and syntenin for the binding to the C terminus of syndecan-2. We fused GST to the intracellular domain (IC) of syndecan-2 to pull-down CASK protein. In the absence of FLAG-syntenin, CASK was pulled down with GST-syndecan-2 IC. However, increasing the amount of FLAG-syntenin in cell lysates suppressed the pull-down of CASK with GST-syndecan-2 in a dose-dependent manner ( Fig. 4g,h ), indicating that syntenin competes with CASK for the binding to syndecan-2. The protein 4.1-binding motif of CASK is involved in spine morphogenesis [27] . Protein 4.1 binds to spectrin [28] and promotes the interaction between spectrin and filamentous actin [28] , [29] ; thus, CASK may act as a linker between transmembrane proteins and the actin cytoskeleton, thereby stabilizing dendritic spines. We therefore sought to determine whether the protein 4.1-binding site of CASK plays a pivotal role in spine synapse morphogenesis. The CASK mutant lacking the protein 4.1-binding motif (CASK Δp4.1 ; Fig. 4c , bottom) lost the ability to increase spine synapse density in Tsc2 +/− neurons ( Fig. 4d ). These results indicate that the protein 4.1-binding site of CASK is required for spine synapse formation in Tsc2 +/− neurons. Taken together, these findings indicate that syntenin may reduce spine synapse density by competing with CASK and preventing it from stabilizing spine morphology via protein 4.1. Binding of syntenin to ephrinB3 increases shaft synapses We previously showed that in Tsc2 +/− neurons, excitatory synapses were rarely located on dendritic protrusions but preferentially localized to dendritic shafts [14] . Syntenin has been demonstrated to be a downstream effector of ephrinB3 (ref. 30 ), which modulates glutamatergic synaptic density [31] , particularly on shaft synapses [32] . To test whether syntenin is involved in excitatory shaft synapse formation, we knocked down syntenin in WT and Tsc2 +/− neurons. Downregulation of syntenin drastically reduced excitatory shaft synapse density in Tsc2 +/− neurons but not in WT neurons ( Fig. 5a ). Next, we examined the involvement of ephrinB3 in the syntenin-mediated shaft synapse formation. We knocked down the endogenous ephrinB3 in Tsc2 +/− hippocampal neurons using ephrinB3 siRNA ( Supplementary Fig. 3a,b ). Eleven days after the ephrinB3 siRNA transfection, we observed a significant reduction in vGlut1 puncta on the dendritic shafts in Tsc2 +/− neurons but not in WT neurons ( Fig. 5b ). EphrinB3 knockdown did not affect spine synapse density in either WT or Tsc2 +/− neurons ( Fig. 5b ). Conversely, overexpression of ephrinB3 increased excitatory shaft synapse density in WT neurons ( Fig. 5c ), and simultaneous expression of syntenin siRNA effectively inhibited this increase ( Fig. 5c ), suggesting that ephrinB3 may regulate shaft synapse density via syntenin. In our experiment, the overexpression of ephrinB3 significantly reduced spine synapse density, which was inconsistent with a previous study [32] . The reason for this difference is unclear, but our overexpression of ephrinB3 plasmid was longer and stronger (10 days under the control of the CAG promoter) than that in the other study [32] (4 days under the control of the cytomegalovirus promoter). Because ephrinB3 regulates synapse density by inhibiting the postsynaptic mitogen-activated protein kinase signalling [31] that is required for increases in spine density [33] , long and strong expression of ephrinB3 might reduce spine synapse density. Future studies will be needed to characterize this mechanism. 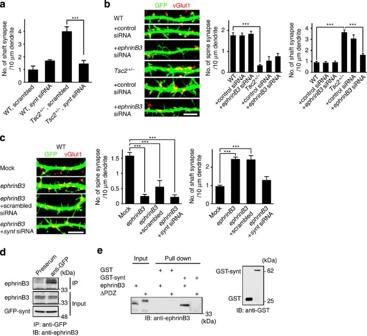Figure 5: Syntenin enhances excitatory shaft synapse density in the downstream of ephrinB3. (a) Quantification of vGlut1 puncta density on dendritic shafts of WT andTsc2+/−neurons transfected with scrambled orsynteninsiRNA (n=500/5/3 (WT, scrambled), 500/5/3 (WT, syntenin siRNA), 1,146/10/5 (Tsc2+/−, scrambled) and 1,034/10/5 (Tsc2+/−, syntenin siRNA) synapses/neurons/experiments, ***P<0.001, two-way ANOVA,post hocTukey test). (b)EphrinB3siRNA decreased shaft synapse formation. (Left)EGFPplasmid and eitherephrinB3siRNA or control siRNA was expressed in WT andTsc2+/−neurons, and the spine and shaft synapse densities were examined. Scale bar, 10 μm. (Right) Quantitative analysis of the data shown in the left panel.EphrinB3siRNA significantly reduced the shaft synapse density inTsc2+/−neurons (n=500/5/3 synapses/neurons/experiments/each condition, ***P<0.001, two-way ANOVA,post hocTukey test). (c) EphrinB3 increased shaft synapse density via syntenin. (Left)EphrinB3was co-expressed in WT neurons withsynteninsiRNA or scrambled siRNA, and the spine and shaft synapse densities were counted. Scale bar, 10 μm. (Right) Quantitative analysis of the data shown in the left panel. EphrinB3-induced shaft synapse increase was inhibited bysynteninsiRNA but not by scrambled siRNA (n=500/5/3 synapses/neurons/experiments/each condition, ***P<0.001, two-way ANOVA,post hocTukey test). (d) Co-immunoprecipitation of ephrinB3 with EGFP-syntenin from HEK293T cells expressing both proteins using anti-GFP antibody. (e) PDZ-dependent binding of syntenin to ephrinB3. EphrinB3- or ephrinB3ΔPDZ-expressing cell lysates were pulled down with GST-syntenin. The precipitates were immunoblotted (IB) with anti-ephrinB3 antibody. Blots ind,eare cropped and full-length blots are presented inSupplementary Fig. 6k,l. All data are presented as mean±s.e.m. Figure 5: Syntenin enhances excitatory shaft synapse density in the downstream of ephrinB3. ( a ) Quantification of vGlut1 puncta density on dendritic shafts of WT and Tsc2 +/− neurons transfected with scrambled or syntenin siRNA ( n =500/5/3 (WT, scrambled), 500/5/3 (WT, syntenin siRNA), 1,146/10/5 ( Tsc2 +/− , scrambled) and 1,034/10/5 ( Tsc2 +/− , syntenin siRNA) synapses/neurons/experiments, *** P <0.001, two-way ANOVA, post hoc Tukey test). ( b ) EphrinB3 siRNA decreased shaft synapse formation. (Left) EGFP plasmid and either ephrinB3 siRNA or control siRNA was expressed in WT and Tsc2 +/− neurons, and the spine and shaft synapse densities were examined. Scale bar, 10 μm. (Right) Quantitative analysis of the data shown in the left panel. EphrinB3 siRNA significantly reduced the shaft synapse density in Tsc2 +/− neurons ( n =500/5/3 synapses/neurons/experiments/each condition, *** P <0.001, two-way ANOVA, post hoc Tukey test). ( c ) EphrinB3 increased shaft synapse density via syntenin. (Left) EphrinB3 was co-expressed in WT neurons with syntenin siRNA or scrambled siRNA, and the spine and shaft synapse densities were counted. Scale bar, 10 μm. (Right) Quantitative analysis of the data shown in the left panel. EphrinB3-induced shaft synapse increase was inhibited by syntenin siRNA but not by scrambled siRNA ( n =500/5/3 synapses/neurons/experiments/each condition, *** P <0.001, two-way ANOVA, post hoc Tukey test). ( d ) Co-immunoprecipitation of ephrinB3 with EGFP-syntenin from HEK293T cells expressing both proteins using anti-GFP antibody. ( e ) PDZ-dependent binding of syntenin to ephrinB3. EphrinB3- or ephrinB3 ΔPDZ -expressing cell lysates were pulled down with GST-syntenin. The precipitates were immunoblotted (IB) with anti-ephrinB3 antibody. Blots in d , e are cropped and full-length blots are presented in Supplementary Fig. 6k,l . All data are presented as mean±s.e.m. Full size image To examine the direct interaction between ephrinB3 and syntenin, we co-immunoprecipitated ephrinB3 with syntenin from HEK293T cells expressing green fluorescent protein (GFP)-syntenin and ephrinB3 ( Fig. 5d ). This binding likely occurred through a PDZ domain because the ephrinB3 mutant lacking the PDZ recognition motif was not associated with syntenin ( Fig. 5e ). Together, these results indicate that syntenin may enhance shaft synapse formation by binding to ephrinB3 through the PDZ domain. Excitatory shaft synapses in Tsc2 +/− neurons are functional In a previous work, to investigate excitatory synaptic transmission in TSC neurons, we systematically investigated the electrophysiological properties of WT and Tsc2 +/− neurons [14] . Unexpectedly, Tsc2 +/− neurons showed sufficient synaptic transmission, with no significant differences in presynaptic or postsynaptic features between WT and Tsc2 +/− neurons. Therefore, we proposed that increased shaft synapses in Tsc2 +/− neurons may functionally compensate for the excitatory synaptic transmission of decreased spine synapses. To test this hypothesis, we reduced shaft synapse density in autaptic WT and Tsc2 +/− neurons by expressing ephrinB3 siRNA, and we electrophysiologically recorded synaptic transmission in these neurons ( Fig. 6a–g ). Although the control siRNA did not affect synaptic transmission in either WT or Tsc2 +/− neurons ( Supplementary Fig. 4a–g ), ephrinB3 siRNA markedly reduced the excitatory postsynaptic current (EPSC) amplitude and miniature EPSC (mEPSC) frequency without changes in the probability of vesicular release in Tsc2 +/− neurons ( Fig. 6a–f ). These data suggest that excitatory synaptic transmission between Tsc 2 +/− neurons is functionally compensated for by increases in the ephrinB3-mediated shaft synapses, leading to the apparent stabilization of synaptic transmission in Tsc2 +/− neurons. Furthermore, we immunostained Tsc2 +/− neurons with anti-GluR1 (GluA1) and vGlut1 antibodies to confirm that postsynaptic receptors are localized next to presynaptic puncta. Indeed, vGlut1 clusters were co-localized with GluA1 puncta on the dendritic shaft of Tsc2 +/− neurons ( Supplementary Fig. 4h ), consistent with the dendritic shaft synapses in Tsc2 +/− neurons being functional. 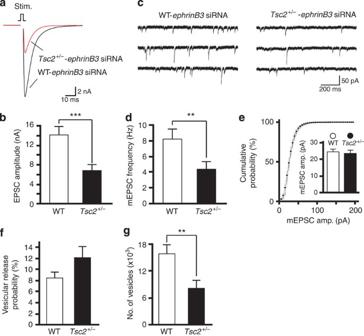Figure 6: Synaptic transmission inTsc2+/−neurons is functionally compensated for by ephrinB3-mediated shaft synapses. (a) Representative evoked EPSC traces obtained from WT andTsc2+/−single hippocampal autaptic neurons treated with ephrinB3 siRNA. The depolarization artefact of the action potential evoked by electrical stimulation (Stim.) was blanked. (b) Mean EPSC amplitude in WT (n=36) andTsc2+/−(n=34) autaptic neurons treated withephrinB3siRNA (***P<0.001). (c) Representative mEPSC traces in WT andTsc2+/−autaptic neurons treated withephrinB3siRNA. (d) Mean mEPSC frequency in WT (n=34) andTsc2+/−(n=35) autaptic neurons treated withephrinB3siRNA (**P<0.01). (e) Cumulative probability plots of the mEPSC amplitude (amp.) in WT (n=34) andTsc2+/−(n=35) autaptic neurons treated withephrinB3siRNA. The inset shows the mean mEPSC amplitude. (f) Mean vesicular release probability in WT (n=30) andTsc2+/−(n=26) autaptic neurons treated withephrinB3siRNA. (g) Mean number of synaptic vesicles in RRP in WT (n=30) andTsc2+/−(n=26) autaptic neurons treated withephrinB3siRNA (**P<0.01). The data were obtained from 21 (WT) and 14 (Tsc2+/−) experiments, respectively. All data are presented as mean±s.e.m. (**P<0.01, ***P<0.001, Student’st-test). Figure 6: Synaptic transmission in Tsc 2 +/− neurons is functionally compensated for by ephrinB3-mediated shaft synapses. ( a ) Representative evoked EPSC traces obtained from WT and Tsc2 +/− single hippocampal autaptic neurons treated with ephrinB3 siRNA. The depolarization artefact of the action potential evoked by electrical stimulation (Stim.) was blanked. ( b ) Mean EPSC amplitude in WT ( n =36) and Tsc2 +/− ( n =34) autaptic neurons treated with ephrinB3 siRNA (*** P <0.001). ( c ) Representative mEPSC traces in WT and Tsc2 +/− autaptic neurons treated with ephrinB3 siRNA. ( d ) Mean mEPSC frequency in WT ( n =34) and Tsc2 +/− ( n =35) autaptic neurons treated with ephrinB3 siRNA (** P <0.01). ( e ) Cumulative probability plots of the mEPSC amplitude (amp.) in WT ( n =34) and Tsc2 +/− ( n =35) autaptic neurons treated with ephrinB3 siRNA. The inset shows the mean mEPSC amplitude. ( f ) Mean vesicular release probability in WT ( n =30) and Tsc2 +/− ( n =26) autaptic neurons treated with ephrinB3 siRNA. ( g ) Mean number of synaptic vesicles in RRP in WT ( n =30) and Tsc2 +/− ( n =26) autaptic neurons treated with ephrinB3 siRNA (** P <0.01). The data were obtained from 21 (WT) and 14 ( Tsc2 +/− ) experiments, respectively. All data are presented as mean±s.e.m. (** P <0.01, *** P <0.001, Student’s t -test). Full size image Furthermore, we noticed that the number of synaptic vesicles in the readily releasable pool (RRP) was significantly reduced by ephrinB3 siRNA in Tsc 2 +/− neurons but not in WT neurons ( Fig. 6g ). In this experiment, we estimated the number of synaptic vesicles in the RRP by simply dividing the hypertonic sucrose-evoked RRP charge by an individual average mEPSC charge; thereby, the RRP charge should involve all synaptic releases from presynaptic terminals projecting to both spine and shaft synapses. Thus, the finding that number of releasable vesicles was reduced by ephrinB3 siRNA in Tsc 2 +/− neurons also implies that dendritic shaft synapses are functional. Because vesicular release probability was unchanged in ephrinB3-knockdown neurons, we believe that presynaptic effects can be excluded. However, because presynaptic development has been shown to be regulated by syntenin [34] , exploring whether presynaptic function is changed in TSC neurons will be the focus of our next study. Syntenin knockout restores spine synapses in Tsc2 +/− neurons To confirm the in vivo function of syntenin using other genetically defined animals, syntenin-floxed mice were generated ( Fig. 7a ). These mice were crossed with αCaMKII Cre mice [35] to obtain CaMKII Cre ;syntenin flox/+ ( syntenin +/− ) mice. Syntenin +/− mice were born in a Mendelian ratio and could not be distinguished from their littermate controls at birth. We further crossed these mice with Tsc2 +/− mice [36] and prepared control (WT, CaMKII Cre or syntenin flox/+ ), syntenin +/− , Tsc2 +/− and Tsc2 +/− ;syntenin +/− mice. We then compared ex vivo dendritic spine morphology of the hippocampal CA1 neurons in each brain slices using DiOlistic labelling. Similar to Tsc2 +/− rat neurons [14] , mouse Tsc2 +/− neurons showed dendritic protrusions that were longer and thinner than those of control neurons ( Fig. 7b,c ). By contrast, genetic hetero-insufficiency of syntenin in Tsc2 +/− neurons increased the width and reduced the length of dendritic protrusions ( Fig. 7b,c ). The protrusion density was also increased in Tsc2 +/− neurons compared with that in control or Tsc2 +/− ;syntenin +/− neurons ( Fig. 7d ). Syntenin +/− neurons showed narrow and thin dendritic protrusions ex vivo ( Fig. 7b,c ). 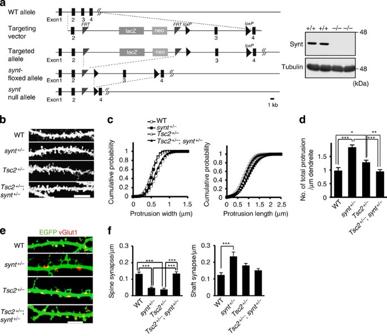Figure 7: Heterozygous knockout ofsynteninrescued spine dysmorphogenesis inTsc2+/−mice. (a) Targeting construct for the generation ofsyntenin-floxed mice. In the targeting vector, exon 3 of thesynteningene was flanked by LoxP sites, indicated with black triangles. The neomycin resistance cassette was surrounded by flippase recognition target sequences, shown as black rectangles (left). Immunoblotting of WT andsynteninknockout brain lysates with anti-syntenin antibody (right). These blots are cropped and full-length blots are presented inSupplementary Fig. 6m. (b) Representative DiI-labelled dendrites of hippocampal CA1 neurons from control,syntenin+/−,Tsc2+/−andTsc2+/−;syntenin+/−mice. Scale bar, 10 μm. (c) Cumulative probability plots of the protrusion widths (left) and lengths (right) as shown inb.Tsc2+/−andsyntenin+/−neurons showed decreased protrusion width (D=0.2706,P<0.001 (Tsc2+/−;syntenin+/−andTsc2+/−),D=0.2417,P<0.001 (Tsc2+/−;syntenin+/−andsyntenin+/−),D=0.4069,P<0.001 (control andTsc2+/−),D=0.3042,P<0.001 (control andsyntenin+/−)) and an increased protrusion length (D=0.0885,P<0.05 (Tsc2+/−;syntenin+/−andTsc2+/−),D=0.1943,P<0.001, (Tsc2+/−;syntenin+/−andsyntenin+/−),D=0.1113,P<0.001 (control andTsc2+/−),D=0.2117,P<0.001 (control andsyntenin+/−)) compared withTsc2+/−;syntenin+/−and control neurons, respectively.Tsc2+/−;syntenin+/−neurons exhibit dendritic protrusions almost identical to those of control neurons. Heterozygous knockout ofsynteninrescued the aberrant protrusion shape inTsc2+/−mice (n=994/10/5 (control), 652/6/4 (syntenin+/−), 1,073/10/5 (Tsc2+/−) and 1,043/10/5 (Tsc2+/−;syntenin+/−) protrusions/neurons/experiments, Kolmogorov–Smirnov test). (d) Quantification of the protrusion density inb.Tsc2+/−andsyntenin+/−neurons exhibited higher protrusion densities thanTsc2+/−;syntenin+/−and control neurons, respectively (*P<0.05, **P<0.01, ***P<0.001, two-way ANOVA,post hocTukey test). (e)Tsc2+/−mouse neurons showed a decrease in excitatory (vGlut1-positive) spine synapse density and an increased in shaft synapse density, and this phenotype was rescued by heterozygous knockout ofsyntenin.Syntenin+/−neurons also showed decreased spine synapse density and increased shaft synapse density. Scale bar, 10 μm. (f) Data quantification ine. All data are presented as mean±s.e.m. (n=500/5/3 synapses/neurons/experiments/each condition, ***P<0.001, two-way ANOVA,post hocTukey test). Figure 7: Heterozygous knockout of syntenin rescued spine dysmorphogenesis in Tsc2 +/− mice. ( a ) Targeting construct for the generation of syntenin -floxed mice. In the targeting vector, exon 3 of the syntenin gene was flanked by LoxP sites, indicated with black triangles. The neomycin resistance cassette was surrounded by flippase recognition target sequences, shown as black rectangles (left). Immunoblotting of WT and syntenin knockout brain lysates with anti-syntenin antibody (right). These blots are cropped and full-length blots are presented in Supplementary Fig. 6m . ( b ) Representative DiI-labelled dendrites of hippocampal CA1 neurons from control, syntenin +/− , Tsc2 +/− and Tsc2 +/− ; syntenin +/− mice. Scale bar, 10 μm. ( c ) Cumulative probability plots of the protrusion widths (left) and lengths (right) as shown in b . Tsc2 +/− and syntenin +/− neurons showed decreased protrusion width ( D =0.2706, P <0.001 ( Tsc2 +/− ; syntenin +/− and Tsc2 +/− ), D =0.2417, P <0.001 ( Tsc2 +/− ; syntenin +/− and syntenin +/− ), D =0.4069, P <0.001 (control and Tsc2 +/− ), D =0.3042, P <0.001 (control and syntenin +/− )) and an increased protrusion length ( D =0.0885, P <0.05 ( Tsc2 +/− ; syntenin +/− and Tsc2 +/− ), D =0.1943, P< 0.001, ( Tsc2 +/− ; syntenin +/− and syntenin +/− ), D =0.1113, P <0.001 (control and Tsc2 +/− ), D =0.2117, P <0.001 (control and syntenin +/− )) compared with Tsc2 +/− ; syntenin +/− and control neurons, respectively. Tsc2 +/− ;syntenin +/− neurons exhibit dendritic protrusions almost identical to those of control neurons. Heterozygous knockout of syntenin rescued the aberrant protrusion shape in Tsc2 +/− mice ( n =994/10/5 (control), 652/6/4 ( syntenin +/− ), 1,073/10/5 ( Tsc2 +/− ) and 1,043/10/5 ( Tsc2 +/− ; syntenin +/− ) protrusions/neurons/experiments, Kolmogorov–Smirnov test). ( d ) Quantification of the protrusion density in b . Tsc2 +/− and syntenin +/− neurons exhibited higher protrusion densities than Tsc2 +/− ; syntenin +/− and control neurons, respectively (* P <0.05, ** P <0.01, *** P <0.001, two-way ANOVA, post hoc Tukey test). ( e ) Tsc2 +/− mouse neurons showed a decrease in excitatory (vGlut1-positive) spine synapse density and an increased in shaft synapse density, and this phenotype was rescued by heterozygous knockout of syntenin . Syntenin +/− neurons also showed decreased spine synapse density and increased shaft synapse density. Scale bar, 10 μm. ( f ) Data quantification in e . All data are presented as mean±s.e.m. ( n =500/5/3 synapses/neurons/experiments/each condition, *** P <0.001, two-way ANOVA, post hoc Tukey test). Full size image Next, we cultured hippocampal neurons from each mouse line and compared the excitatory spine and shaft synapse densities among control, syntenin +/− , Tsc2 +/− and Tsc2 +/− ; syntenin +/− neurons. Mouse Tsc2 +/− neurons showed a reduced spine synapse density and an increased shaft synapse density, whereas the heterozygous knockout of syntenin reversed these abnormalities in Tsc2 +/− neurons ( Fig. 7e,f ). Mouse s yntenin +/− neurons again showed a decrease in spine synapse density ( Fig. 7e,f ), as observed in syntenin-knockdown rat WT neurons ( Fig. 2h,i ). To confirm these results, we electrophysiologically analysed synaptic properties of mouse control, syntenin +/− , Tsc2 +/− and Tsc2 +/− ;syntenin +/− neurons ( Supplementary Fig. 5 ). Similar to rat Tsc2 +/− neurons, mouse Tsc2 +/− neurons showed no significant changes compared with control neurons in evoked EPSC amplitude, mEPSC amplitude, mEPSC frequency, vesicular release probability and number of releasable vesicles. Tsc2 +/− ;syntenin +/− neurons also showed electrophysiological properties similar to those of control, suggesting that syntenin reduction may change the spine/shaft synapse ratio in Tsc2 +/− neurons without affecting overall excitatory synaptic transmission. However, we found that the mEPSC frequency was significantly reduced in syntenin +/− neurons compared with that in Tsc2 +/− ;syntenin +/− neurons. Notwithstanding, evoked EPSC amplitude, mEPSC amplitude and other presynaptic functions were unchanged between syntenin +/− and Tsc2 +/− ;syntenin +/− neurons. The reason for this decrease in syntenin +/− neurons is unclear, but it may reflect the reduction in spine synapse density without increases in shaft synapse density in syntenin +/− neurons ( Fig. 7e,f ). Thus, genetic knockout of syntenin can restore both dendritic spine and shaft synapse densities in Tsc2 +/− mice. The present study suggests a novel mechanism for the regulation of excitatory spine and shaft synapse morphogenesis via Rheb-syntenin signalling. We also show that this mechanism is dysregulated in TSC neurons. 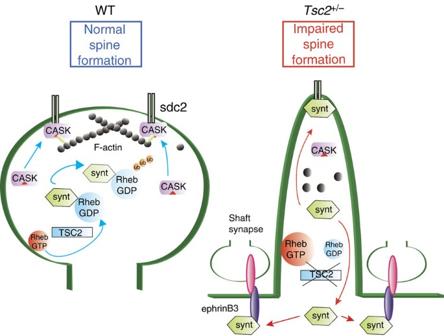Figure 8: Proposed model for the role of Rheb and syntenin in spine and shaft synapse formation. During normal development, Tsc2 (tuberin) converts Rheb-GTP into inactive Rheb-GDP. Rheb-GDP binds to syntenin, thereby promoting syntenin degradation. This decrease in syntenin levels may facilitate the association of CASK with syndecan-2 (sdc2) and the formation of spinal F-actin, leading to normal spine development (left, WT). However,Tsc2disruption in tuberous sclerosis increases Rheb-GTP, which rescues syntenin from proteasomal destruction. Accumulated syntenin may inhibit the binding of CASK to sdc2 and promote its binding to ephrinB3, resulting in impaired spine morphogenesis and enhanced shaft synapse formation (right,Tsc2+/−). Figure 8 summarizes our working model in which Rheb and syntenin are essential regulators of the formation of spine and shaft synapses. During normal development, the hamartin/tuberin complex inactivates Rheb-GTPase, which associates with syntenin and triggers the subsequent degradation of the protein complex by the proteasome. Upon Rheb activation through Tsc mutation(s), Rheb dissociates from syntenin and binds to FKBP38 (ref. 37 ) and/or PLD1 (ref. 38 ), resulting in the activation of mTORC1. Accumulated syntenin binds to syndecan-2 in dendritic protrusions, thereby competitively excluding CASK. Because CASK links syndecan-2 with the actin cytoskeleton via protein 4.1 (ref. 16 ), the elimination of CASK may destabilize the spine structure. In addition, syntenin binds to ephrinB3 in dendritic shafts and enhances excitatory shaft synapse formation. Our results indicate that the association between syndecan-2 and CASK is crucial for normal spine synapse development, and the disruption of this interaction by syntenin may cause abnormalities in dendritic spine and shaft synapses. Figure 8: Proposed model for the role of Rheb and syntenin in spine and shaft synapse formation. During normal development, Tsc2 (tuberin) converts Rheb-GTP into inactive Rheb-GDP. Rheb-GDP binds to syntenin, thereby promoting syntenin degradation. This decrease in syntenin levels may facilitate the association of CASK with syndecan-2 (sdc2) and the formation of spinal F-actin, leading to normal spine development (left, WT). However, Tsc2 disruption in tuberous sclerosis increases Rheb-GTP, which rescues syntenin from proteasomal destruction. Accumulated syntenin may inhibit the binding of CASK to sdc2 and promote its binding to ephrinB3, resulting in impaired spine morphogenesis and enhanced shaft synapse formation (right, Tsc2 +/− ). Full size image Consistent with a human Golgi study [12] , mouse models of TSC have demonstrated dendritic spine abnormalities [13] , [39] . In particular, Tavazoie et al. [13] showed that Tsc1 deficiency in cultured hippocampal slices led to decreased spine density, increased spine length and head width. These findings are somewhat different from our observations (decreased spine synapse density, increased protrusion length and decreased protrusion width in dissociated Tsc2 +/− neurons). This discrepancy may reflect differences in culture conditions (slice culture versus dissociated culture) and/or neuronal maturation. However, the common finding is that these spine abnormalities were not restored by inhibition of mTORC1. We previously found that suppression of Rheb-GTPase activity with farnesyl transferase inhibitors almost completely rescued spine synapse formation [14] . Thus, a non-canonical pathway such as this Rheb-syntenin signalling may participate in some of the symptomatic manifestations in TSC [40] , [41] , [42] . Indeed, knockdown and knockout of brain syntenin restored contextual fear discrimination deficits in Tsc2 +/− rats and mice, respectively (unpublished data). In addition, to confirm our findings using human neurons, we will generate mutations in Tsc gene in human-induced pluripotent stem cells for differentiation into excitatory neurons. These future results may provide new mechanistic insights into the pathogenesis of neurological symptomatic manifestations in TSC patients. Furthermore, development of a method to control Rheb activity in living neurons may strengthen a direct link between the Rheb-syntenin signalling and spine formation. We show that increased syntenin diminished spine synapse density in TSC neurons, whereas a previous study demonstrated that syntenin overexpression in WT neurons did not reduce spine synapse density [30] . This discrepancy may be caused by the use of different antibodies to detect presynaptic terminals; we immunolabelled only excitatory synapses with anti-vGlut1, whereas Xu et al. [30] used an anti-synapsin antibody that reacts with both excitatory and inhibitory terminals. Because inhibitory synapses were also increased in TSC neurons (unpublished data), the use of an anti-synapsin antibody might produce different results from this study. The other difference between this study and that by Xu et al. [30] is in the mEPSC frequency in ephrinB3-reduced neurons. We found no significant change in the mEPSC frequency in ephrinB3-knockdown WT neurons ( Fig. 6d and Supplementary Fig. 4d ), whereas Xu et al. [30] showed a clear decrease in mEPSC frequency in ephrinB3-deficient neurons [30] . This discrepancy may be because of the differences in neuronal maturation. We used cultured hippocampal neurons at DIV 14–23, whereas Xu et al. [30] euthanized P12 mice for electrophysiology. Excitatory synapses translocate from dendritic shafts (shaft synapses) to spines (spine synapses) during neuronal development [43] . We used mature neurons with fewer shaft synapses, which are the main targets of regulation by ephrinB3 (ref. 32 ). This may explain why ephrinB3 knockdown failed to reduce synaptic transmission in this study. Reducing the syntenin levels in WT neurons also decreased the spine synapse density ( Fig. 2h,i ). Thus, the deviation of syntenin levels from a narrow physiological range may disrupt spine synapse formation. In contrast to Tsc2 +/− neurons, however, syntenin +/− neurons did not show increased shaft synapse density ( Fig. 7f ), suggesting that syntenin reduction may affect only spine synapses. How the reduction in syntenin levels decreases spine synapse density remains unclear; however, it is noteworthy that syntenin associates with multiple proteins, such as adhesion molecules (SynCAM [44] , neurexin and neurofascin [45] ) or cytoplasmic proteins (PICK1; ref. 46 ). The absence of these associations may contribute to impaired spine formation. It is possible that such distinct syntenin function regulates dendritic spinogenesis in different ways. Clarification of this mechanism will be the next step in understanding the multiple functions of syntenin. CASK is also a scaffold protein that interacts with >20 of binding partners through its PDZ domain. In postsynaptic neurons, both syntenin and CASK can bind to syndecan-2, which regulates dendritic spine formation [26] . We show that the increase in syntenin levels may impair spine synapse morphogenesis in Tsc2 +/− neurons. Such synaptic abnormalities in TSC neurons may be a cause of mental retardation and/or refractory epilepsy in early childhood, called West syndrome [5] . In addition, CASK gene mutations cause intractable epilepsy and intellectual disability in infancy [47] , called Ohtahara syndrome [48] . Ohtahara syndrome often evolves into West syndrome, therefore these two syndromes are both classified as ‘epileptic encephalopathy’. Thus, the increases in syntenin levels and the CASK mutations may cause related neurodevelopmental disorders, suggesting that the two proteins functionally compete against each other. Here, we focused on the contributions of postsynaptic syntenin and CASK to the control of spine formation; however, both proteins are also localized to presynaptic terminals and bind to β-neurexin [49] , [50] . To examine the presynaptic effects of Tsc2 mutations on excitatory synapse formation, we compared the size of vGlut1 puncta in WT-WT synapses and Tsc2 +/− -WT synapses; however, we found no significant differences (0.11±0.013 mm 2 for WT and 0.10±0.011 for Tsc2 +/− boutons). Because syntenin knockdown in postsynaptic TSC neurons results in spine synapse formation with presynaptic TSC neurons, spine formation may be regulated by the postsynaptic balance between syntenin and CASK rather than by presynaptic effects. Future studies are needed to characterize the effects of presynaptic syntenin and CASK on spine and shaft synapse formation. In this study, we found that Rheb interacted with syntenin and formed a novel part of the TSC–Rheb pathway, which may help us to better understand the pathophysiology of neurological symptoms in TSC. Several preclinical studies and early human case reports have demonstrated that mTORC1 inhibitors such as sirolimus or everolimus are useful for treating seizures [39] , [51] , [52] , [53] , [54] , whereas more recent prospective trials have shown that benefits could not be demonstrated when seizure frequency was analysed as a secondary outcome measure [55] , [56] . Moreover, 10–20% of TSC patients showed exacerbation of seizures after everolimus treatment, even in the clinical trial that demonstrated the efficacy of everolimus [57] . Thus, in addition to mTORC1 inhibitors, new approaches for the treatment of neurological symptoms in TSC patients are needed to improve not only seizure control but also cognitive function and patient quality of life. Because Rheb expression is regulated by neuronal activity [58] , Rheb-syntenin signalling may be involved in activity-dependent learning and memory processes. Appropriate modulation of this signalling pathway can be required for normal cognitive function. Thus, the Rheb-syntenin pathway may also be a therapeutic target for relieving TSC and other cognitive disorders involving abnormalities of spine and shaft synapses. Antibodies and reagents Antibodies used for western blotting are summarized in Supplementary Table 1 . Rapamycin, MG132 and lactacystin were purchased from LKT Laboratories, Millipore and the Peptide Institute, respectively. The siRNAs used in this study are summarized in Supplementary Table 2 . Oligonucleotides were synthesized and duplexed by Invitrogen (Stealth, syntenin and syndecan-2 ) and Dharmacon (Accell, ephrinB3 ). Their suppressive activities were confirmed in rat neurons and HEK293T cells using immunostaining and western blotting, respectively. Animals The Eker ( Tsc2 +/ – ) and WT genotypes were determined using PCR [59] . Syntenin-floxed mice were obtained from the Knock-Out Mouse Project ( www.komp.org ; project no. CSD26463). CaMKII Cre mice [35] were obtained from European Mouse Mutant Archive. Tsc2 +/ – mice were generated previously [36] Mice were maintained on a C57BL/6 background. All of the animal experiments were approved by the Animal Care and Use Committees of the Tokyo Metropolitan Institute of Medical Science and Fukuoka University. Molecular cloning and plasmid construction The full-length of rat Rheb was subcloned into a yeast expression vector, pPC97 (ref. 60 ), in a fusion complex with the GAL4 DNA-binding domain. This construct was transformed in yeast strain PCY2 (ref. 60 ). Transformants were selected on leucine-deficient (Leu − ) medium and subsequently transformed with an oligo(dT)-primed rat hippocampal cDNA library subcloned into pPC86 (ref. 61 ). Positive colonies were selected on triple-deficient plates (Leu − , Trp − and adenine − ) and were assayed for β-galactosidase activity. Their plasmids were isolated and transformed into Escherichia coli . The E. coli clones containing the pPC86 construct were rescued and their plasmids were isolated and sequenced. For expression in primary neurons, COS-7 cells and HEK293T cells, rat Rheb , syntenin and syndecan-2 cDNAs were cloned into the EGFP-C3, ECFP-C3 and pEF-FLAG vectors, respectively. Rat CASK and Rheb cDNAs were cloned into ECFP-C3 and pEF-FLAG, respectively. EphrinB3 cDNA was cloned into pCAG. The syntenin Δ N(1–115) mutant was generated using PCR from rat syntenin cDNA. Using the QuikChange Site-Directed Mutagenesis Kit (Stratagene), Rheb mutants (D60I, T38M/D60I, I39K/D60I and Q64V), syntenin mutants (mPDZ1, mPDZ2, ΔC(278–300), ΔC(289–300), ΔC(289–294) and ΔC(295–300)), a CASK mutant (Δ4.1) and an ephrinB3 mutant (ΔPDZ) were generated from WT Rheb , syntenin , CASK and ephrinB3 , respectively [27] , [49] , [62] . The siRNA-resistant forms of the syntenin mutants and ephrinB3 were generated through the introduction of silent mutations in the syntenin and ephrinB3 siRNA target sequences, respectively. Immunoprecipitation Rat brains, COS-7 cells and HEK293T cells were homogenized with lysis buffer (20 mM Tris-HCl (pH 8.0), 0.15 M NaCl, 1 mM EDTA, 1% Triton X-100, protease inhibitor cocktail tablet (Roche) and 1 mM phenylmethylsulfonyl fluoride). The homogenates were centrifuged to obtain clear protein extracts. Anti-syntenin (goat, Santa Cruz Biotechnology), anti-GFP (rabbit, Invitrogen) or anti-FLAG (mouse, Sigma-Aldrich) antibodies were added to the protein extracts on ice for 1 h, and the mixtures were incubated overnight at 4 °C with packed protein G Sepharose (GE Healthcare). The precipitated immune complex was boiled in SDS sample buffer and analysed using western blotting with anti-Rheb (rabbit, CST), anti-FLAG (mouse, Sigma-Aldrich), anti-GFP (rabbit, Invitrogen) or anti-ephrinB3 (rabbit, Invitrogen) antibodies [63] . All representative western blots included in the manuscript are shown as full scans in Supplementary Fig. 6 . Recombinant protein expression and pull-down assay For the bacterial expression of recombinant GST-tagged syntenin and the syntenin mutants, the corresponding sequences were cloned into the pGEX-4T2 vector (GE Healthcare) and expressed in BL21(DE3) cells. Each GST-fused syntenin protein was purified with glutathione beads (GE Healthcare). To examine the binding between Rheb and syntenin, the same amount of purified GST-syntenin (WT or mutant) was first attached to glutathione beads and then incubated with cell extracts expressing various versions of enhanced green fluorescent protein (EGFP)-tagged Rheb overnight at 4 °C. To determine whether the nucleotide-binding state of Rheb affects the binding of syntenin to the IC of syndecan-2, the purified GST-syndecan-2 IC protein was first attached to glutathione beads and then incubated with cell extracts expressing FLAG-tagged syntenin and either EGFP-Rheb D60I or EGFP-Rheb Q64V overnight at 4 °C. To examine the binding between syntenin and ephrinB3, the purified GST-syntenin was first incubated with cell extracts expressing ephrinB3 or ΔPDZ overnight at 4 °C. In all pull-down experiments, the beads were washed with lysis buffer and boiled in SDS sample buffer. The precipitates were analysed using western blotting with anti-GFP, anti-FLAG or anti-ephrinB3 antibodies. All representative western blots included in the manuscript are shown as full scans in Supplementary Fig. 6 . Cell culture and transfection All cells were cultured at 37 °C and 5% CO 2 . Neuronal cultures were prepared from hippocampi at embryonic day 19–21 for Eker rats and at postnatal day 0–1 for control (WT, CaMKII Cre or syntenin flox/+ ), syntenin +/− , Tsc2 +/− and Tsc2 +/− ; syntenin +/− mice. Cells were plated at a density of 5,400 cells per cm 2 onto polyethyleneimine-coated dishes. Primary cultures were maintained in neurobasal medium supplemented with B27, gentamicin and GlutaMAX. The neurons were transfected with expression plasmids and/or siRNAs at DIV 11–12 using Lipofectamine 2000 (Invitrogen) [64] . The transfection of ephrinB3 siRNA into primary neurons was performed according to the Thermo Scientific Dharmacon Accell siRNA Delivery Protocol (Thermo Scientific). HEK293T and COS-7 cells were obtained from R. Takahashi (Riken) and T. Haga (University of Tokyo), respectively. Both cells were plated at 70–80% confluence onto polyethyleneimine-coated dishes and cultured in DMEM supplemented with 10% fetal bovine serum. Cells were transfected with plasmids using Lipofectamine 2000 (Invitrogen) [63] . To quantify the proteasome degradation of Rheb and syntenin proteins, Rheb- and syntenin-coexpressing COS-7 cells were untreated or treated with 20 μM MG132 for 20 h. Cultured hippocampal neurons were treated with 0.5 μM lactacystin for 2 days (DIV 17–19) or 100 nM MG132 for 1 day (DIV 18–19). Cell lysates were immunoblotted with anti-GFP. Immunostaining Rat cultured hippocampal neurons were fixed with 4% paraformaldehyde, blocked, permeabilized with BL solution (3% normal goat serum or 3% bovine serum albumin with 0.1% Triton X-100 in PBS) and incubated overnight at 4 °C with one of the following primary antibodies: anti-syntenin (mouse, Santa Cruz Biotechnology), anti-GFP (chicken, Millipore), anti-vGlut1 (guinea pig, Millipore) or anti-ephrinB3 (rabbit, Invitrogen). The immunoreactivity was visualized using species-specific, fluorochrome-conjugated secondary antibodies. For spine and shaft synapse density analysis, dendrites were chosen randomly and their lengths were measured in two-dimensional projection of three-dimensional image stacks. Spines were defined as any protrusions from the dendritic shaft <8 μm in length [32] . The number of vGlut1 puncta on spine and shaft synapses of the dendritic segment is determined by counting the number of vGlut1 puncta that partially overlap with the GFP-positive shaft or spines. Any vGlut1 puncta that are not touching the GFP-positive dendrite are not included. Image acquisition and quantification Confocal images of neurons were obtained using a Zeiss 63 × lens (numerical aperture 1.4) with sequential acquisition settings at the resolution of the confocal microscope (512 × 512 pixels). Each image was a composite constructed from a series of images captured throughout the z axis of each cell. The parameters of each composite image were optimized for the particular lens and pinhole setting. Identical confocal microscope settings were maintained for all scans in each experiment. All morphometric analyses and quantifications were performed using MetaMorph image analysis software (Universal Imaging). For the spine morphology studies, individual dendritic protrusions were manually traced, and the maximum length and head width of each dendritic protrusion were measured and recorded in Microsoft Excel. To measure the average pixel fluorescence intensity of syntenin, the neurons were carefully traced and the background intensity was subtracted from the intensity in the traced regions. Neurons were selected blindly based on the GFP or MAP2 fluorescence. Autaptic culture Astrocytes were obtained from cerebral cortices of newborn (P0) ICR mice (Kyudo). Cerebral cortices were removed from the brains, placed in cold Hank’s Balanced Saline Solution (Invitrogen) and dissociated using 0.05% trypsin-EDTA (Wako). The cells were plated in plating medium composed of Dulbecco’s modified Eagle medium with GlutaMax and pyruvate (DMEM, Invitrogen) supplemented with 10% fetal bovine serum (Invitrogen) and 0.1% MITO+ Serum Extender (BD Biosciences) in 75 cm 2 culture flasks (250 ml, BD Falcon). The next day, the culture flask was gently rinsed once with plating medium to remove non-adherent cells. After 2 weeks, when the glial cells had almost reached confluence, microglia and other small cells were isolated and removed by tapping the culture flask several times. The remaining astrocytes adhered to the bottom of the culture bottle were subsequently trypsinized and plated onto microdot-coated coverslips (see above) in the plating medium at a density of 6,000 cells per cm 2 . Once microislands were uniformly established on the coverslip, within a week, an antimitotic agent (8 μM 5-fluoro-2′-deoxyuridine (Sigma-Aldrich) and 20 μM uridine (Sigma-Aldrich)) was added to curtail glial proliferation and maintain the purity of the microisland cultures. The microisland culture plates were established a few days before the neuronal cultures. The autaptic cultures of rat E18–19 and mouse P0–1 hippocampal neurons were generated [65] , [66] , [67] . Briefly, CA1-CA3 hippocampi were isolated and enzymatically dissociated in papain (2 units per ml, Worthington) in DMEM for 60 min at 37 °C. The dissociated hippocampal neurons were plated at a density of 1,500 cells per cm −2 onto the above astrocyte island plates. Before plating the dissociated hippocampal neurons, the astrocyte-conditioned media was replaced with Neurobasal-A medium (Invitrogen) supplemented with 2% B27 supplement (Invitrogen) and GlutaMax. The medium was not changed during the neuronal culture periods. Electrophysiology All synaptic recordings were undertaken on autaptic cultures after genotyping. In all cases, the synaptic responses from autaptic neurons were recorded in the whole-cell configuration under the voltage-clamp mode at a holding potential (V h) of −70 mV (MultiClamp 700B, Molecular Devices) and room temperature. The patch pipette resistance was 3–6 MΩ, and the series resistance was compensated by 70–90%. The α-amino-3-hydroxy-5-methyl-4-isoxazolepropionic acid (AMPA) receptor-mediated evoked glutamatergic synaptic transmission was recorded in response to an action potential elicited by a brief (2 ms) somatic depolarization pulse (to +0 mV) from the patch pipette. Spontaneous glutamatergic mEPSCs were recorded in the presence of 0.5 μM tetrodotoxin. The size of the RRP of synaptic vesicles was estimated using a synaptic transient charge elicited by a 10-s application of 0.5 M sucrose. The number of synaptic vesicles in the RRP was subsequently calculated by dividing the RRP charge by the individual average mEPSC charge. The vesicular release probability was calculated as the ratio of the charge of the evoked EPSC to the RRP charge successfully obtained from the same neuron. The synaptic responses were recorded at a sampling rate of 20 kHz and filtered at 10 kHz. The data were excluded from the analysis if a leak current >300 pA was observed. The template for the mEPSC data analysis was set as a rise time constant of 0.5 ms, a decay time constant of 4 ms, a baseline of 5 ms, and a template length of 10 ms. The data were analysed offline using Axograph X 1.2 software (AxoGraph Scientific). Recordings of synaptic responses were performed at DIV 14–23 and DIV 13–16 from rat and mouse neurons, respectively. The standard extracellular solution contained (in mM) NaCl 140, KCl 2.4, HEPES 10, glucose 10, CaCl 2 2 and MgCl 2 1, with pH 7.4 and an adjusted osmotic pressure of 315–320 mOsm. Patch pipettes were filled with an intracellular solution containing (in mM) K-gluconate 146.3, MgCl 2 0.6, ATP-Na 2 4, GTP-Na 2 0.3, phosphocreatine 12, EGTA 1 and HEPES 17.8, as well as creatine phosphokinase 50 U ml −1 (pH 7.4). Hypertonic solutions for determining the RRP size were prepared by adding 0.5 M sucrose to the standard extracellular solution. The extracellular solutions were applied using a fast-flow application system (Warner Instruments). Each flow pipe had a diameter of 430 μm, ensuring that the solution was applied to all parts of an autaptic neuron on the astrocytic microisland (300 × 300 μm). This configuration was necessary to facilitate the application of sucrose to induce the release of RRP vesicles from all nerve terminals of the recorded neuron. All chemicals were purchased from Sigma-Aldrich unless otherwise specified. DiOlistic labelling Six- to eight-week-old mice were deeply anaesthetized with 0.1 mg kg −1 phenobarbital and perfused transcardially with 0.1 M phosphate buffer, followed by 50 ml of 2% paraformaldehyde. The brains were dissected and postfixed in the same fixative for 4 h. Subsequently, sagittal brain sections were obtained using a vibratome and collected in PBS. Twenty-five milligrams of gold particles (Bio-Rad) were coated with 7.0 mg of the lipophilic dye DiI (Invitrogen) and injected into Tefzel tubing, which was subsequently cut into bullets. These particles were delivered DiOlistically at 80 p.s.i. using a Helios gene-gun system (Bio-Rad). The slices were fixed again with 4% PFA at 4 °C for 1 h and mounted on slides in VectaShield Mounting Medium (Vector Laboratories). Statistical analysis Statistical analyses were performed using Student’s t -test, two-way analysis of variance with proper post hoc tests or the Kolmogorov–Smirnov test, as specified in each figure legend. Differences were considered significant when P <0.05. How to cite this article: Sugiura, H. et al. Rheb activation disrupts spine synapse formation through accumulation of syntenin in tuberous sclerosis complex. Nat. Commun. 6:6842 doi: 10.1038/ncomms7842 (2015).